Unc5C and DCC act downstream of Ctip2 and Satb2 and contribute to corpus callosum formation The pyramidal neurons of the mammalian neocortex form two major types of long-range connections—corticocortical and cortico-subcortical. The transcription factors Satb2 and Ctip2 are critical regulators of neuronal cell fate that control interhemispheric versus corticofugal connections respectively. Here, we investigate the axon guidance molecules downstream of Satb2 and Ctip2 that establish these connections. We show that the expression of two Netrin1 receptors- DCC and Unc5C is under direct negative regulation by Satb2 and Ctip2, respectively. Further, we show that the Netrin1–Unc5C/DCC interaction is involved in controlling the interhemispherical projection in a subset of early born, deep layer callosal neurons. The neocortex is the neural substrate of our higher cognitive abilities, helping us perceive, understand and react to the environment. Such a formidable task is made possible by the staggering number of neurons that constitute the neocortex forming functional connections both within the neocortex as well as with other targets in the central nervous system. Such long-range connections are crucial for brain function and the efficient integration and exchange of information. The long-range connections of the neocortex can be broadly classified into two types: interhemispheric connections versus corticofugal connections. While most deeper layer neurons (layer V–VI) make corticofugal connections, upper layer neurons (II–III) and some neurons of layer V connect the two hemispheres of the telencephalon. Although both laterally and medially projecting layer V neurons are born at the same time, laterally projecting neurons extend an axon ~2 days before the medially projecting layer V neurons [1] . The corpus callosum (CC) is the primary conduit for transmission and coordination of information between neurons of the two cerebral hemispheres. Evolutionarily, the mammalian neocortex has undergone a substantial increase in the proportion of upper layer neurons suggesting that the corresponding increase in corticocortical connections is one of the primary reasons for the increase in the cognitive abilities witnessed through mammalian evolution [2] , [3] , [4] . It is hence no surprise that malformation or agenesis of the CC can lead to severe cognitive disabilities [5] . Although it has been well established that neurons form connections through specific and predetermined trajectories in the brain in response to several guidance cues present in the environment, our understanding of how cellular identities govern the appropriate responses of axons to these guidance cues and hence direct the establishment of these precise connections remains incomplete, more so for forebrain structures such as the neocortex [1] . Two genes, Satb2 and Ctip2, have been shown in recent years to orchestrate important and mutually exclusive genetic programs that establish corticocortical versus corticofugal connections, respectively [6] , [7] , [8] . While Satb2, a matrix attachment region (MAR) interacting protein has been shown to be indispensable for the formation of the CC, Ctip2 on the other hand is required for the fasciculation and pathfinding of subcortically projecting neurons [6] , [9] . Interestingly, the deletion of Satb2 in the cortex leads to an ectopic upregulation of Ctip2 in upper layer neurons, with a corresponding misrouting of callosally projecting neurons to subcortical targets [7] , [8] . Thus, in normal development, Satb2 overrides the Ctip2 driven molecular pathway in order to establish interhemispheric projections versus corticofugal projections. In this study, we investigated the downstream molecular events in this Satb2— Ctip2 interaction. We identified that two Netrin1 receptors, DCC and Unc5C , are controlled by both Satb2 and Ctip2. Unc5C and DCC play important roles in guiding commissural axons in various systems [10] , [11] , [12] , [13] , [14] , [15] . DCC can mediate an attractive response to a Netrin1 source, while Unc5C, in a DCC-dependent or -independent manner, has been shown to mediate a repulsive response [11] , [12] , [15] , [16] , [17] , [18] . Here, we show that Ctip2 and Satb2 negatively regulate Unc5C and DCC , respectively. This in turn mediates a differential response of neocortical axons to Netrin1. High levels of Unc5C expression, and low levels of DCC expression, instruct neurons to project through the CC, since in the absence of either Unc5C or Netrin1 , callosal axons misproject to subcortical targets, mimicking the effect of Satb2 mutation. In contrast, inactivation of Ctip2 and DCC , or the restoration of Unc5C in Satb2 mutants, can partially restore CC formation. Thus, a dynamic regulation of Unc5C and DCC by Ctip2 and Satb2 paves the way for the appropriate formation of interhemispheric and corticofugal neocortical projections, at least for a subset of deep layer callosal neurons. Unc5C expression requires Satb2 In order to identify molecules downstream of Satb2 that control CC formation, we investigated changes in the expression of a variety of axon guidance molecules in the Satb2 −/− mutants. We assumed that such molecules should be downregulated in Satb2 -mutant cortex and that their expression should be confined to callosal neurons (Satb2 positive), while being excluded from corticofugal neurons (Ctip2 positive). Among others tested, the expression of the Netrin1 receptor, Unc5C, satisfied these two criteria. Unc5C expression was previously shown to be downregulated in Satb2 −/− mutants [7] , [19] . Here, in situ hybridization against the Unc5C messenger RNA (mRNA) showed a complete loss of Unc5C from the Satb2 −/− cortical plate, with only expression in the subplate remaining ( Fig. 1a ). Further, Unc5C has a very dynamic expression pattern during cortical development. At E14.5 Unc5C is predominantly expressed in the subplate. At E18.5, the expression of Unc5C in the cortical plate reaches a very high level and demonstrates a high-lateral to low-medial gradient ( Fig. 1a,b ). 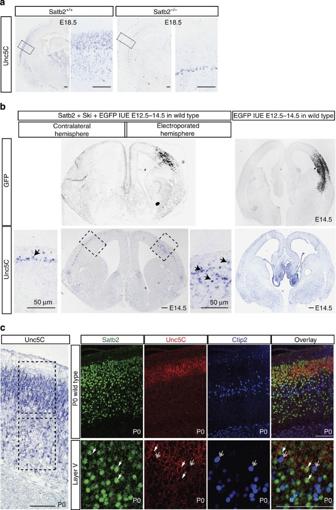Figure 1: Unc5C is expressed by callosally projecting Satb2-positive neurons and Satb2 regulatesUnc5Cexpression. (a)Unc5CmRNA expression in wild-type andSatb2−/−-mutant mice at E18.5. In sections ofSatb2−/−-mutant brains,Unc5Ccontinues to be expressed in only the subplate, but is absent in other cortical layers. (b)Unc5Cexpression in E14.5 wild-type embryos in cells that were electroporated at E12.5 withSatb2/Ski/EGFPorEGFPcontrol. GFP IHC depicts the region electroporated.Unc5C in situhybridization shows additional ectopic expression ofUnc5Cwithin cells electroporated withSatb2/Skiapart from the expression in the subplate seen in the contralateral hemisphere or in the control electroporation. (c)Unc5CmRNA expression with respect to Satb2 and Ctip2-expressing cells through immunofluorescence/fluorescence ISH in P0 wild-type cortex. High magnification of P0 wild-type cortex shows thatUnc5Cis expressed primarily in the upper layers but also in a subset of cells in the deep layers—layer V (boxed regions)Unc5CmRNA expression coincides with the expression of Satb2 and is excluded from Ctip2-expressing cells. Layer V expression ofUnc5Cis restricted to cells expressing Satb2 (arrows) and absent in Ctip2-positive cells (double arrowheads). Scale bar, 100 μm, unless specified differently in the figure. Figure 1: Unc5C is expressed by callosally projecting Satb2-positive neurons and Satb2 regulates Unc5C expression. ( a ) Unc5C mRNA expression in wild-type and Satb2 −/− -mutant mice at E18.5. In sections of Satb2 −/− -mutant brains, Unc5C continues to be expressed in only the subplate, but is absent in other cortical layers. ( b ) Unc5C expression in E14.5 wild-type embryos in cells that were electroporated at E12.5 with Satb2/Ski/EGFP or EGFP control. GFP IHC depicts the region electroporated. Unc5C in situ hybridization shows additional ectopic expression of Unc5C within cells electroporated with Satb2/Ski apart from the expression in the subplate seen in the contralateral hemisphere or in the control electroporation. ( c ) Unc5C mRNA expression with respect to Satb2 and Ctip2-expressing cells through immunofluorescence/fluorescence ISH in P0 wild-type cortex. High magnification of P0 wild-type cortex shows that Unc5C is expressed primarily in the upper layers but also in a subset of cells in the deep layers—layer V (boxed regions) Unc5C mRNA expression coincides with the expression of Satb2 and is excluded from Ctip2-expressing cells. Layer V expression of Unc5C is restricted to cells expressing Satb2 (arrows) and absent in Ctip2-positive cells (double arrowheads). Scale bar, 100 μm, unless specified differently in the figure. Full size image To test whether ectopic and premature expression of Satb2 can induce Unc5C expression, we performed in utero electroporation of Satb2 and Ski expressing plasmids into the lateral ventricle at E12.5 and analysed the brains at E14.5. Satb2 requires Ski as a cofactor for recruiting chromatin remodelling complexes and thus silencing its targets [20] . This experiment induced ectopic expression of Unc5C in the cells electroporated with Satb2 compared with a control construct ( Fig. 1b ). To test our hypothesis that Unc5C is expressed by callosally projecting Satb2-positive cells and absent in Ctip2-positive cells, we combined in situ hybridization (ISH) using a probe against Unc5C and immunohistochemistry (IHC) using antibodies against Satb2 and Ctip2. Unc5C mRNA is expressed predominantly in upper layers and weakly in deeper layers. Since combining ISH and IHC requires the omission of proteinase K from the protocol, a physical limitation to the extent of probe penetration is an unavoidable drawback. Thus, even though in conventional ISH, Unc5C expression is seen in both upper and deeper layers, with FISH the expression was detected in separate experiments. We observed that Unc5C and Ctip2 were not expressed in the same cells in most cases whereas Unc5C and Satb2 were usually co-expressed. Even in layer V, Unc5C and Satb2 were co-expressed but neither was expressed in Ctip2-positive cells ( Fig. 1c ). This indicates that Satb2 could also repress Ctip2 in deep layer neurons, in addition to the previously reported repression in upper layer neurons ( Supplementary Fig. 1A,B ). Unc5C is directly repressed by Ctip2 Since Unc5C and Ctip2 are not co-expressed, we hypothesized that Unc5C expression could be negatively regulated by Ctip2. To investigate this, we examined whether Unc5C expression would be restored in Satb2 −/− ; Ctip2 −/− double mutants. We observed an increase of Unc5C expression in Satb2 −/− ; Ctip2 −/− mutant cortex as compared with Satb2 −/− mutants. In Ctip2 −/− single mutants we did not detect significant changes in Unc5C expression compared with controls ( Fig. 2a ). In all further experiments, wild type, Satb2 heterozygous, Ctip2 heterozygous and Satb2/Ctip2 compound heterozygous embryos have all been referred to interchangeably as controls. 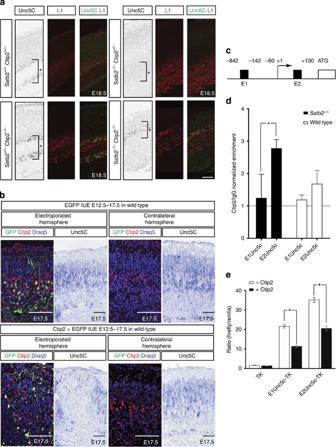Figure 2: Ctip2 directly repressesUnc5Cexpression. (a) Immunohistochemical staining against Unc5C and L1. Unc5C expression is absent inSatb2−/−brains when compared with wild-type andCtip2−/−brains. The expression of Unc5C is restored inSatb2−/−;Ctip2−/−double-mutant brains. (b)Unc5Cexpression in E17.5 wild-type embryos in cells electroporated at E12.5 withCtip2/EGFPorEGFPcontrol within the electroporated as well as contralateral hemisphere. Subsequent section stained for GFP, Ctip2, Draq5 (a nuclear marker) IHC.Unc5CmRNA expression is lost in the region electroporated withCtip2when compared with either the control electroporation or the corresponding region in the contralateral hemisphere. (c) Scheme showing the two regions in theUnc5Cpromoter where Ctip2 was predicted to bind. (d) ChIP from P0 cortex of wild-type andSatb2−/−mutants show that Ctip2 binds to theUnc5Cpromoter region. 2.78±0.2722-fold enrichment for E2 compared with 1.23±0.73 for E1 inSatb2−/−,n=3,P-value=0.027 (Student’st-test) and 1.67±0.42-fold enrichment for E2 compared with 1.18±0.14 for E1 in wild typen=4, NS. (e) Luciferase assay to demonstrate that Ctip2 binds toUnc5Cgenomic region and represses its expression. In the presence of full-length Ctip2, 1.9- and 1.7-fold decrease in luminescence ratio was observed in case of E1 and E2, respectively. E1 and E2 being two putative Ctip2-binding sites. All *P-values were ≤0.05, Student’st-testn=3. Scale bar, 100 μm. Figure 2: Ctip2 directly represses Unc5C expression. ( a ) Immunohistochemical staining against Unc5C and L1. Unc5C expression is absent in Satb2 −/− brains when compared with wild-type and Ctip2 −/− brains. The expression of Unc5C is restored in Satb2 −/− ;Ctip2 −/− double-mutant brains. ( b ) Unc5C expression in E17.5 wild-type embryos in cells electroporated at E12.5 with Ctip2/EGFP or EGFP control within the electroporated as well as contralateral hemisphere. Subsequent section stained for GFP, Ctip2, Draq5 (a nuclear marker) IHC. Unc5C mRNA expression is lost in the region electroporated with Ctip2 when compared with either the control electroporation or the corresponding region in the contralateral hemisphere. ( c ) Scheme showing the two regions in the Unc5C promoter where Ctip2 was predicted to bind. ( d ) ChIP from P0 cortex of wild-type and Satb2 −/− mutants show that Ctip2 binds to the Unc5C promoter region. 2.78±0.2722-fold enrichment for E2 compared with 1.23±0.73 for E1 in Satb2 −/− , n =3, P -value=0.027 (Student’s t -test) and 1.67±0.42-fold enrichment for E2 compared with 1.18±0.14 for E1 in wild type n =4, NS. ( e ) Luciferase assay to demonstrate that Ctip2 binds to Unc5C genomic region and represses its expression. In the presence of full-length Ctip2, 1.9- and 1.7-fold decrease in luminescence ratio was observed in case of E1 and E2, respectively. E1 and E2 being two putative Ctip2-binding sites. All * P -values were ≤0.05, Student’s t -test n =3. Scale bar, 100 μm. Full size image This result indicated that in Satb2 −/− mutants, the downregulation of Unc5C could be the result of the ectopic upregulation of Ctip2 . To test this hypothesis, we overexpressed Ctip2 in the cortex. An EGFP -expression plasmid was electroporated either alone or with the Ctip2 expression plasmid in wild-type E12.5 embryos and the brains were harvested at E17.5. Ctip2 expression was validated in HEK293T cells ( Supplementary Fig. 2A ) and a confocal maximum Z-projection image for the electroporated region also confirmed the expression of Ctip2 in a large population of cortical cells ( Supplementary Fig. 2B ). Subsequent sections were labelled with a probe against Unc5C mRNA. A decrease in Unc5C expression was observed in Ctip2 overexpressing cells within the electroporated cortical region, as compared with the contralateral hemisphere ( n =3) or EGFP -alone electroporated brains ( n =2, Fig. 2b ). Next, we investigated whether Ctip2 directly represses Unc5C expression. An in silico search revealed two putative Ctip2-binding sites in the Unc5C promoter, that we designated E1 and E2 (−842 to −142 and −60 to +100) upstream of the transcription-initiation site ( Fig. 2c ). Chromatin immunoprecipitation (ChIP) from wild-type and Satb2 −/− cortices followed by quantitative real time polymerase chain reaction, showed that Ctip2 binds strongly to the E2 but not the E1 Unc5C promoter region. Satb2 −/− cortices were used as a means of enriching for Ctip2-positive cells in the cortex ( Fig. 2d , 2.78±0.2722-fold enrichment for E2 compared with 1.23±0.73 for E1 in Satb2 −/− , n =3, P -value=0.027 (Student’s t -test) and 1.67±0.42-fold enrichment for E2 compared with 1.18±0.14 for E1 in wild type, n =4, NS). To confirm this result we performed an in vitro luciferase assay. In these experiments, the same two Unc5C upstream genomic regions E1 and E2 were inserted into a plasmid encoding the luciferase gene and transfected into cells with a plasmid encoding Ctip2 . We observed a decrease in the activity of the Unc5C promoter by ~1.9-fold and 1.7-fold, in the case of E1 and E2 respectively, when Ctip2 was co-transfected ( Fig. 2e , both P -values <0.05, Student’s t -test, n =3). These results indicate that Ctip2 can directly repress Unc5C transcription. Partial restoration of the CC in Satb2 −/− ;Ctip2 −/− mutants Others and we have previously shown that the deletion of Satb2 results in the ectopic upregulation of Ctip2 and misprojection of callosal axons laterally [7] , [8] . Since Satb2 and Ctip2 regulate divergent genetic programs, that control the formation of interhemispheric versus corticofugal projections, we investigated whether downregulating Ctip2 in the Satb2 −/− cortex could restore CC formation. We analysed Satb2 −/− ; Ctip2 −/− double-mutant animals for the presence of the CC. To visualize callosal axons, we introduced a plasmid coding for Venus-green fluorescent protein (GFP) in neocortical cells by in utero electroporation at E12.5 and harvested the brains at E18.5. We found that while in Satb2 −/− animals, no cortical axons approached or even turned towards the dorsal midline, in Satb2 −/− ; Ctip2 −/− compound mutants, GFP-positive axons approached, crossed the midline and invaded the contralateral cortex. It is noteworthy though that the number of crossing axons that projected into the contralateral hemisphere were fewer when compared with that seen in wild-type and Ctip2 −/− littermates ( Fig. 3a ). The results were quantified by measuring the fluorescent area of the fibres projecting medially with respect to the fluorescent area of the electroporated region in the cortex ( Supplementary Fig. 3 ). To rule out the possibility of axonal outgrowth defects in Satb2 -negative neurons as a cause for the lack of extension of the axons contralaterally, we performed an in vitro axon outgrowth assay, but did not observe an axonal outgrowth deficit in Satb2- deficient neurons ( Supplementary Fig. 4 ). Another possibility was that the axons were indirectly affected due to changes in the formation of midline guidepost structures in the Satb2 mutant and Satb2 −/− ;Ctip2 −/− double mutants. To examine this, we stained for midline guidepost cells with calretinin and glial fibrillary acidic protein ( Supplementary Fig. 5 ). We did not detect any differences in the size or morphology of midline structures between the different genotypes suggesting that Satb2 -deficient neurons are defective in axonal targeting and not outgrowth or midline crossing. 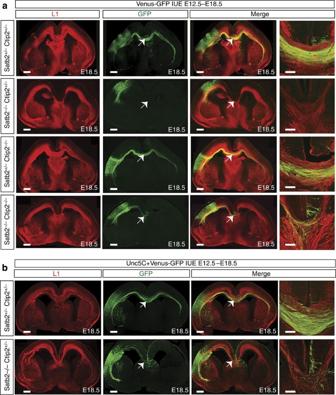Figure 3: The CC is partially restored inSatb2−/−mutants by deletingCtip2or by overexpressingUnc5C. (a) Images with higher magnification of the midline show a series of experiments, whereinVenus-GFPwas electroporated into the developing cortex at E12.5 and the brains harvested and analysed at E18.5. Electroporation ofVenus-GFPshows a normal CC in wild-type andCtip2−/−embryos.Satb2−/−-mutant brains clearly demonstrate a complete absence of callosal fibres, wherein no fibres could be seen approaching the midline. Partial rescue of the CC could be seen inSatb2−/−;Ctip2−/−compound mutants. Fibres manage to reach and cross the midline (arrows). The sections have been subjected to immunohistochemical staining for the neural cell adhesion molecule L1 and for GFP. (b) Images show the result ofUnc5C/EGFPoverexpression in wild-type andSatb2−/−-mutant cortex. Overexpression ofUnc5CinSatb2−/−partially restores the CC where axons of electroporated neurons reach and cross the midline (arrow). Normally projecting callosal axons were observed in the control cortex. Scale bar, 450 μm for low-magnification images and 100 μm for high-magnification images. Figure 3: The CC is partially restored in Satb2 −/− mutants by deleting Ctip2 or by overexpressing Unc5C . ( a ) Images with higher magnification of the midline show a series of experiments, wherein Venus-GFP was electroporated into the developing cortex at E12.5 and the brains harvested and analysed at E18.5. Electroporation of Venus-GFP shows a normal CC in wild-type and Ctip2 −/− embryos. Satb2 −/− -mutant brains clearly demonstrate a complete absence of callosal fibres, wherein no fibres could be seen approaching the midline. Partial rescue of the CC could be seen in Satb2 −/− ; Ctip2 −/− compound mutants. Fibres manage to reach and cross the midline (arrows). The sections have been subjected to immunohistochemical staining for the neural cell adhesion molecule L1 and for GFP. ( b ) Images show the result of Unc5C/EGFP overexpression in wild-type and Satb2 −/− -mutant cortex. Overexpression of Unc5C in Satb2 −/− partially restores the CC where axons of electroporated neurons reach and cross the midline (arrow). Normally projecting callosal axons were observed in the control cortex. Scale bar, 450 μm for low-magnification images and 100 μm for high-magnification images. Full size image Restoring Unc5C expression in Satb2 −/− partially rescues the CC Since the Satb2 −/− ;Ctip2 −/− double mutants showed a partial rescue of callosal crossing fibres and an increased Unc5C expression compared with single mutants, we tested whether we could rescue callosal fibres in Satb2 −/− mutants by overexpressing Unc5C . An Unc5C -expressing plasmid was co-expressed with Venus-GFP at E12.5 and compared with Venus-GFP expression alone in Satb2 −/− as well as control brains. We observed that axons of the Unc5C electroporated neurons in the Satb2 −/− cortex extended medially, and crossed the midline ( n =3). This rescue was again only partial as fewer axons crossed the midline compared with that in the control animals ( Fig. 3b ). Electroporation of only Venus-GFP in Satb2 −/− embryos served as a negative control where no callosally extending fibres were observed ( Fig. 3a ). The extent of callosal midline crossing with electroporation of Unc5C was comparable with the partial rescue obtained in Satb2 −/− ;Ctip2 −/− double mutants at E12.5 ( Fig. 3a,b , Supplementary Fig. 3 ). Interestingly, Unc5C could not restore the callosal fibres when overexpressed at E14.5 ( Supplementary Fig. 6A ). Neocortical callosal axons are repelled by Netrin1 Unc5C has been shown to be a receptor for the secreted ligand Netrin1, mediating long range repulsive signalling [12] , [16] . Since we observed that the formation of callosal projections depended upon the presence of Unc5C expression, we tested whether these Unc5C-positive callosally projecting neurons were also responsive to Netrin1. To test this, we devised a slice culture system where wild-type embryos were co-electroporated with either Unc5C and EGFP ( Fig. 4a ) or only EGFP ( Fig. 4b ) at E12.5 and harvested at E16.5. Slices prepared from these brains were cultured for 3 days in vitro and Netrin1-soaked agarose beads were placed in the midline at the position where callosal fibres cross. If the Unc5C -positive callosal axons were responsive to the repulsive Netrin1 signal, then they would be prevented from crossing the midline upon encountering the ligand in their trajectory. When Unc5C -positive fibres encountered Netrin1-soaked beads in the midline, they were repelled and did not cross the midline. Instead they misprojected ventrally or dorsally within the ipsilateral hemisphere showing an avoidance behaviour towards the beads. Conversely, when these Unc5C -positive axon fibres encountered bovine serum albumin (BSA)-soaked beads, they were unaffected and continued in their trajectory, crossing the midline and entering the contralateral hemisphere ( Fig. 4a ). This experiment indicated that Unc5C -expressing cortical neurons are indeed repelled by a Netrin1 source. By expressing only EGFP in cortical neurons, we tested our hypothesis that if callosal fibres express Unc5C endogenously, then they would also be repelled from a Netrin1 source. Again, these fibres failed to cross the midline upon encountering Netrin1, whereas BSA-coated beads posed no hindrance to the midline crossing ( Fig. 4b ). 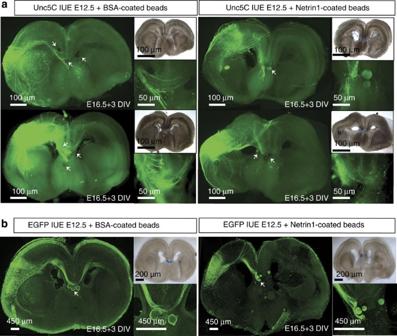Figure 4: Netrin1 repels Unc5C-positive neocortical axons. Images showing the axonal trajectory of neurons electroporated withUnc5C(a) orEGFP(b) on encountering neutral BSA-coated beads (arrows) or Netrin1-coated beads (arrows). Unc5C-positive fibres are unaffected by BSA-coated beads, placed along the midline, and continue along their initial trajectory to project into the contralateral hemisphere. Unc5C-positive fibres, upon encountering a Netrin1 source in the midline show clear repulsive behaviour with fibres projecting either dorsal or ventral to their initial path, but none continuing into the contralateral hemisphere. Wild-type axons electroporated with onlyEGFP(with endogenous Unc5C) are unaffected by the BSA beads and are repelled by the Netrin1 beads similar to theUnc5Coverexpressing axons. Scale bar specified in the figure. Figure 4: Netrin1 repels Unc5C-positive neocortical axons. Images showing the axonal trajectory of neurons electroporated with Unc5C ( a ) or EGFP ( b ) on encountering neutral BSA-coated beads (arrows) or Netrin1-coated beads (arrows). Unc5C-positive fibres are unaffected by BSA-coated beads, placed along the midline, and continue along their initial trajectory to project into the contralateral hemisphere. Unc5C-positive fibres, upon encountering a Netrin1 source in the midline show clear repulsive behaviour with fibres projecting either dorsal or ventral to their initial path, but none continuing into the contralateral hemisphere. Wild-type axons electroporated with only EGFP (with endogenous Unc5C) are unaffected by the BSA beads and are repelled by the Netrin1 beads similar to the Unc5C overexpressing axons. Scale bar specified in the figure. Full size image Satb2-positive axons misproject in Netrin1 and Unc5C mutants Since Unc5C is expressed in Satb2-positive neurons ( Fig. 1c ), and their axons are repelled by Netrin1 in vitro ( Fig. 4 ), we asked whether Netrin1 deletion would have any effect on axons of these neurons in vivo . In the developing telencephalon, Netrin1 is expressed in the basal ganglia and ventral midline [14] , [21] . We reasoned that the source of Netrin1 in the basal ganglia might normally repel the axons of Satb2 -positive/ Unc5C -positive neurons from the internal capsule. We hypothesized that Satb2-positive neurons would misproject to subcortical targets in Netrin1- deficient brains. To test this hypothesis, we placed crystals of the lipophilic tracer DiI at the cerebral peduncle of E17.5 Netrin1 hypomorph and wild-type brains to retrogradely trace the neurons that project subcortically. After staining these sections with an antibody against Satb2, we counted the proportion of DiI-positive retrogradely labelled neurons that were also Satb2 positive ( Fig. 5a ). We observed that the proportion of Satb2-positive DiI-labelled cells representing the proportion of Satb2-positive, subcortically projecting neurons, almost doubled in Netrin1 hypomorph brains compared with their wild-type littermates ( Fig. 5b , 15.36% in wild type compared with 27.33% in Netrin1 hypomorph, P -value=0.011, Student’s t -test, n =3). 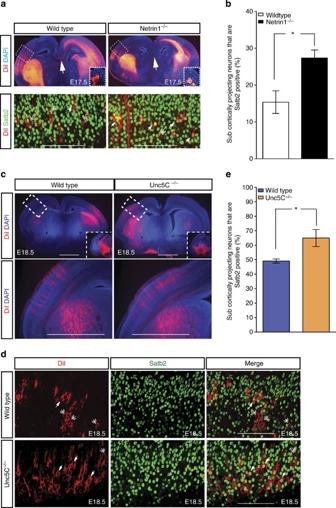Figure 5: Axons of Satb2 neurons are similarly misrouted to subcortical targets inNetrin1andUnc5C−/−mutants. (a) Retrograde labelling of subcerebrally projecting neurons by placing crystals of DiI in the cerebral peduncle of wild-type andNetrin1−/−brains. The smaller inset image shows the respective position of the crystal placement. Retrogradely labelled DiI-positive cells were colocalized with Satb2 in wild-type andNetrin1-mutant brains. Arrows point towards double-positive cells while double arrows highlight single DiI-positive cells. (b) Quantification of the percentage of DiI-positive cells that are Satb2 positive; 15.36% in wild type versus 27.33% in E17.5Netrin1mutant, *P-value=0.011 (Student’st-test),n=3. Error bars represent s.e.m. (c) Crystals of the lipophilic tracer DiI were placed in the cerebral peduncle of wild-type andUnc5C−/−brains to retrogradely label cortical neurons projecting subcerebrally. The smaller inset images show the location of the crystals placed in the cerebral peduncle. Higher magnification image of the boxed region show layer V neurons back-labelled in the cortex. (d) Colocalization of DiI-positive and Satb2-positive cells in the neocortex. Arrows indicate double-positive cells, while double arrows indicate single DiI-positive cells. Scale bar, 100 μm. (e) Quantification of the proportion of subcortically projecting neurons that are Satb2 positive; 49.10% in wild type versus 64.98% in E18.5Unc5C−/−; *P-value=0.0286 (Student’st-test),n=3. Error bars represent s.e.m. Figure 5: Axons of Satb2 neurons are similarly misrouted to subcortical targets in Netrin1 and Unc5C −/− mutants. ( a ) Retrograde labelling of subcerebrally projecting neurons by placing crystals of DiI in the cerebral peduncle of wild-type and Netrin1 −/− brains. The smaller inset image shows the respective position of the crystal placement. Retrogradely labelled DiI-positive cells were colocalized with Satb2 in wild-type and Netrin1 -mutant brains. Arrows point towards double-positive cells while double arrows highlight single DiI-positive cells. ( b ) Quantification of the percentage of DiI-positive cells that are Satb2 positive; 15.36% in wild type versus 27.33% in E17.5 Netrin1 mutant, * P -value=0.011 (Student’s t -test), n =3. Error bars represent s.e.m. ( c ) Crystals of the lipophilic tracer DiI were placed in the cerebral peduncle of wild-type and Unc5C −/− brains to retrogradely label cortical neurons projecting subcerebrally. The smaller inset images show the location of the crystals placed in the cerebral peduncle. Higher magnification image of the boxed region show layer V neurons back-labelled in the cortex. ( d ) Colocalization of DiI-positive and Satb2-positive cells in the neocortex. Arrows indicate double-positive cells, while double arrows indicate single DiI-positive cells. Scale bar, 100 μm. ( e ) Quantification of the proportion of subcortically projecting neurons that are Satb2 positive; 49.10% in wild type versus 64.98% in E18.5 Unc5C −/− ; * P -value=0.0286 (Student’s t -test), n =3. Error bars represent s.e.m. Full size image We also tested whether Unc5C ablation in neocortical neurons would cause a similar effect. In contrast to the acallosal Netrin1 hypomorph, Unc5C mutants display callosal fibres crossing the midline. We therefore tested whether some axons that would normally project to the CC are redirected to the internal capsule in the Unc5C mutant. We performed similar DiI retrograde-labelling experiments in Unc5C −/− brains and counted the number of Satb2-positive cells projecting to the internal capsule ( Fig. 5c,d ). We found that the proportion of Satb2-positive, subcortically projecting cells was 16% higher in the Unc5C mutants compared with wild-type littermate brains ( Fig. 5e ; 49.1% in wild type versus 64.98% in Unc5C −/− brains, P -value=0.0286, Student’s t -test n =3). Therefore, although callosal axons cross the midline in the Unc5C mutant, more Satb2-positive axons project to the internal capsule in both these mutants. This finding indicates that a Netrin1–Unc5C interaction plays an important role in determining the choice of axonal target projection (medially versus laterally), in a cell autonomous manner. Satb2 is a direct repressor of DCC transcription Since restoring the expression of Unc5C in Satb2 −/− mutants lead to only a partial rescue of the CC, we tested whether additional axon guidance molecules in this pathway that are important in CC formation displayed altered expression in Satb2 −/− brains. Like Unc5C, DCC is also a receptor for Netrin1, but has been shown to mediate axonal attraction [22] . We performed immunohistochemical staining and in situ hybridization for DCC in wild type as well as Satb2 −/− cortices at E18.5. Both, DCC protein and mRNA expression was upregulated in Satb2 −/− brains as compared with wild-type littermates ( Fig. 6a ). In contrast, no changes in DCC expression were observed between the control and Ctip2 −/− or between the Satb2 −/− ;Ctip2 −/− double mutant and Satb2 −/− single mutant indicating that Ctip2 did not effect DCC expression ( Supplementary Fig. 7 ). 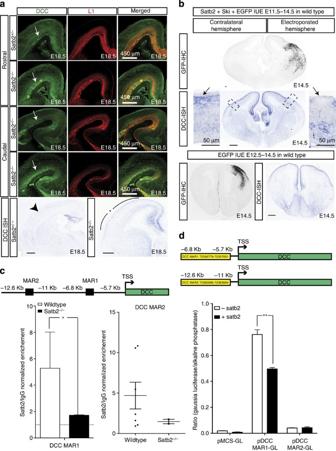Figure 6:DCCis negatively regulated by Satb2 and is upregulated in theSatb2−/−cortex. (a) Immunohistochemical staining for DCC in rostral and caudal sections shows an upregulation of DCC expression inSatb2−/−mutant brains as compared with wild-type littermates. Arrows point to the region of altered DCC expression between wild-type andSatb2−/−sections. ISH reflects an upregulation ofDCCin E18.5Satb2−/−cortex when compared withSatb2heterozygous brains. (b) Series of images showDCCexpression in E14.5 wild-type embryos in cells electroporated with eitherSatb2/Ski/EGFPat E11.5 or withEGFPalone at E12.5. GFP IHC delineates the region electroporated.DCCISH demonstrates a downregulation ofDCCmRNA within cells electroporated withSatb2/Skicompared withDCCexpression in the contralateral hemisphere, or in the control electroporation. (c) Schematic diagram showing two putative binding MAR sites for Satb2 upstream of theDCCtranscription-initiation site. ChIP from P0 cortices showed a 5.27±2.75-fold enrichment inn=6 wild-type compared with 1.72±0.015 inn=2Satb2−/−mutants forDCCMAR1, *P-value=0.025 (Student’st-test) and forDCCMAR2,n=7 wild-type showed a range of 0.91–10.83-fold enrichment with an average of 4.69±4.38, as compared with 1.47±0.39 inn=2Satb2−/−mutants,P-value=0.10 (Student’st-test). (d) Luciferase assay to demonstrate that Satb2 binds to theDCCgenomic region and represses its expression. In the presence of full-lengthSatb2,DCCMAR1 showed a 1.5-fold decrease in luminescence ratio whileDCCMAR2 did not shown any change (Student’st-test, **P-value=0.0035). Scale bar, 100 μm, unless specified differently in the figure. Figure 6: DCC is negatively regulated by Satb2 and is upregulated in the Satb2 −/− cortex. ( a ) Immunohistochemical staining for DCC in rostral and caudal sections shows an upregulation of DCC expression in Satb2 −/− mutant brains as compared with wild-type littermates. Arrows point to the region of altered DCC expression between wild-type and Satb2 −/− sections. ISH reflects an upregulation of DCC in E18.5 Satb2 −/− cortex when compared with Satb2 heterozygous brains. ( b ) Series of images show DCC expression in E14.5 wild-type embryos in cells electroporated with either Satb2/Ski/EGFP at E11.5 or with EGFP alone at E12.5. GFP IHC delineates the region electroporated. DCC ISH demonstrates a downregulation of DCC mRNA within cells electroporated with Satb2/Ski compared with DCC expression in the contralateral hemisphere, or in the control electroporation. ( c ) Schematic diagram showing two putative binding MAR sites for Satb2 upstream of the DCC transcription-initiation site. ChIP from P0 cortices showed a 5.27±2.75-fold enrichment in n =6 wild-type compared with 1.72±0.015 in n =2 Satb2 −/− mutants for DCC MAR1, * P -value=0.025 (Student’s t -test) and for DCC MAR2, n =7 wild-type showed a range of 0.91–10.83-fold enrichment with an average of 4.69±4.38, as compared with 1.47±0.39 in n =2 Satb2 −/− mutants, P -value=0.10 (Student’s t -test). ( d ) Luciferase assay to demonstrate that Satb2 binds to the DCC genomic region and represses its expression. In the presence of full-length Satb2 , DCC MAR1 showed a 1.5-fold decrease in luminescence ratio while DCC MAR2 did not shown any change (Student’s t -test, ** P -value=0.0035). Scale bar, 100 μm, unless specified differently in the figure. Full size image In the wild-type cortex, DCC demonstrated a very dynamic pattern of expression. In contrast to Unc5C expression, DCC mRNA expression is high in the cortical plate at E14.5 ( Fig. 6b ) and below detection levels at E18.5. Only a low level of DCC protein expression was observed in the white matter at E18.5 ( Fig. 6a ). In order to investigate if Satb2 could regulate DCC expression, we overexpressed Satb2 and Ski prematurely in wild-type cortex at E11.5 and analysed the brains for DCC expression at E14.5. Again, Ski was co-electroporated to enable Satb2 to recruit the transcription repressor complex. At E14.5, since there are few endogenous Satb2-positive cells in the cortex and since DCC expression is high in the cortical plate, we assumed that any alteration in DCC expression would be observable. In this experiment, DCC expression was significantly lower in the electroporated region compared with the non-electroporated hemisphere ( n =2). In contrast, EGFP electroporation alone did not alter the expression of DCC ( n =2, Fig. 6b ). To investigate whether Satb2 could directly control DCC expression, we performed ChIP assays for two putative Satb2-binding sites (MAR1 and MAR2) upstream of the DCC transcription-initiation site ( Fig. 6c ). These regions are AT rich and could therefore serve as Satb2-binding sites. We observed a significant enrichment of the region more proximal to the TSS (MAR1) in wild-type tissue as compared with Satb2 -mutant tissue, which served as the negative control (5.27±2.75-fold enrichment in n =6 wild type compared with 1.72±0.015 in n =2 Satb2 −/− mutants, P -value=0.025, Student’s t -test). In contrast, enrichment for the second MAR region (MAR2) was highly variable indicating that Satb2 might bind very weakly to this promoter region ( n =7 wild type showed a range of 0.91–10.83-fold enrichment with an average of 4.69±4.38, as compared with 1.47±0.39 in n =2 Satb2 −/− mutants, P -value=0.10, Student’s t -test). To further investigate the functional significance of this MAR binding, we cloned the two genomic regions, DCC MAR1 and DCC MAR2, into a Gaussia Luciferase vector and transfected them into COS cells either in the presence or absence of Satb2 . DCC MAR1 (chromosome 18 72356779–72357851) showed a 1.5-fold decrease in transcription levels when co-expressed with Satb2 ( Fig. 6d , n =3, P -value=0.0035, Student’s t -test, n =3). DCC MAR2 (chromosome 18 72362066–72363664) did not show any change in transcription levels upon Satb2 co-expression ( Fig. 6d , n =3, P -value=0.742, Student’s t -test, n =3). Taken together, these findings suggest that Satb2 can directly repress DCC expression and might be another factor influencing corticocortical versus cortico-subcortical axon targeting choice. Downregulating DCC in Satb2 −/− partially rescues the CC To test the hypothesis that DCC upregulation contributed to the misrouting of callosal axons in Satb2-deficient brains, we tested whether downregulating DCC in the Satb2 mutant could restore callosal projections. We tested the downregulation efficiency of four different small hairpin RNA (shRNA) constructs by transfecting DCC shRNA or the scrambled shRNA together with a DCC expression plasmid in HEK cells and checking protein levels by western blot ( Supplementary Fig. 8 ). Based on these experiments, we selected two DCC shRNA constructs (clone 2 and 4) and co-electroporated them with Venus-GFP at E12.5 in Satb2 −/− and wild-type cortices. While callosal axons crossed the midline in wild-type brains electroporated with either the DCC shRNA or the scrambled shRNA, no midline crossing fibres were observed when scrambled shRNA was electroporated in Satb2 −/− brains ( n =2). In contrast, neurons electroporated with DCC shRNA in the Satb2 −/− cortex now extended towards and crossed the midline ( n =3, Fig. 7 , Supplementary Fig. 3 ). The rescue was, however, again only partial. 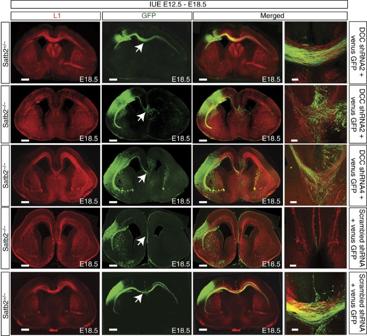Figure 7: DownregulatingDCCin theSatb2−/−cortex leads to a partial rescue of the CC. Images show a series of experiments, whereinin uteroelectroporation was done at E12.5 and the brains harvested and analysed at E18.5.In uteroelectroporation ofDCCshRNA andVenus-GFPdo not seem to have a major effect on the formation of the CC in wild-type embryos.In uteroelectroporation of two differentDCCshRNAs (shRNA2 and shRNA4) along withVenus-GFPshows a reproducible partial rescue of the CC inSatb2−/−embryos.In uteroelectroporation of a scrambled shRNA andVenus-GFPcannot rescue the CC inSatb2−/−embryos. Arrows point towards the dorsal midline. Scale bar, 450 μm for low-magnification images and 100 μm for high-magnification images. Figure 7: Downregulating DCC in the Satb2 −/− cortex leads to a partial rescue of the CC. Images show a series of experiments, wherein in utero electroporation was done at E12.5 and the brains harvested and analysed at E18.5. In utero electroporation of DCC shRNA and Venus-GFP do not seem to have a major effect on the formation of the CC in wild-type embryos. In utero electroporation of two different DCC shRNAs (shRNA2 and shRNA4) along with Venus-GFP shows a reproducible partial rescue of the CC in Satb2 −/− embryos. In utero electroporation of a scrambled shRNA and Venus-GFP cannot rescue the CC in Satb2 −/− embryos. Arrows point towards the dorsal midline. Scale bar, 450 μm for low-magnification images and 100 μm for high-magnification images. Full size image Together, these results indicate that Satb2 directly represses the expression of DCC and that an upregulation of DCC in the Satb2 −/− cortex could contribute to the lack of callosal axons crossing the midline. It is also interesting to note that downregulation of DCC at later stages of development (E14.5), could not restore callosal projections, indicating that only a population of deep layer neurons contributed to forming the restored projections ( Supplementary Fig. 6B ). In order to test whether the extent of CC restoration in Satb2 mutants could be enhanced, we simultaneously inactivated DCC and overexpressed Unc5C in Satb2 mutants. Surprisingly, in these experiments, we did not detect any CC restoration ( Supplementary Fig. 9 ). Satb2/Ctip2 control of DCC/Unc5C regulates only DL callosal projections Callosal neurons are a heterogeneous population of neurons [23] . With respect to the molecular mechanisms described here, deep neocortical layers, born before E14.5 are dependent upon the Netrin1/Unc5C/DCC pathway. However, upper layer neurons, born after E14.5 probably require pathway(s) other than Netrin1/Unc5C/DCC. The lack of a complete restoration of the CC in Satb2 mutants after Unc5C upregulation or DCC downregulation, questioned the extent of the cell autonomous contribution of Satb2 to CC formation. We therefore electroporated a Satb2 expression plasmid together with EGFP into Satb2 −/− brains at E12.5. At E18.5, we observed that although the electroporated neurons in the Satb2 −/− mutants were able to form a CC, the rescue of the CC was again only partial, similar to the rescues obtained in case of either the Satb2 −/− ;Ctip2 −/− double mutants, Unc5C overexpression or DCC downregulation in the Satb2 −/− mutants ( n =2, Fig. 8 , Supplementary Fig. 3 ). A similar principal seems to be underlying all of these scenarios as Satb2 upon ectopic overexpression in wild-type cortices can lead to Unc5C overexpression ( Fig. 1b ) and DCC downregulation ( Fig. 6b ). We also tested the ability of the electroporated Satb2 in repressing Ctip2 and found an absence of Ctip2 protein from the electroporated cells ( Supplementary Fig. 10 ). 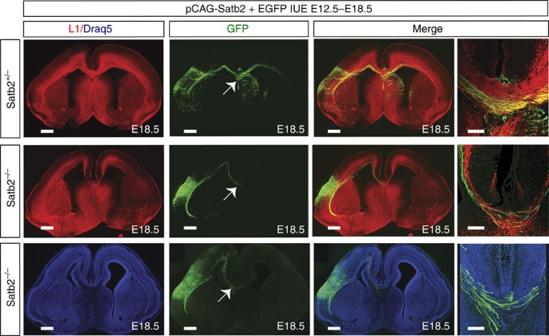Figure 8:Satb2electroporation inSatb2−/−cortex partially rescues the CC. In uteroelectroporation of plasmids encoding forSatb2andEGFPin wild-type andSatb2−/−embryos at E12.5, harvested at E18.5 followed by immunohistochemical staining for the neuronal adhesion molecule L1, show a partial rescue of the CC inSatb2−/−mutants. Alternatively, sections were counter stained with the far-red nuclear marker Draq5. Arrows indicate fibres crossing the midline. Scale bar, 450 μm for low-magnification images and 100 μm for high-magnification images. Figure 8: Satb2 electroporation in Satb2 −/− cortex partially rescues the CC. In utero electroporation of plasmids encoding for Satb2 and EGFP in wild-type and Satb2 −/− embryos at E12.5, harvested at E18.5 followed by immunohistochemical staining for the neuronal adhesion molecule L1, show a partial rescue of the CC in Satb2 −/− mutants. Alternatively, sections were counter stained with the far-red nuclear marker Draq5. Arrows indicate fibres crossing the midline. Scale bar, 450 μm for low-magnification images and 100 μm for high-magnification images. Full size image Again, we did not observe any rescue of the CC upon overexpression of Satb2 at later stages (E14.5, Supplementary Fig. 6C ). The information processing ability of the nervous system relies heavily on the precise establishment of neuronal connections. The expression of Satb2 or Ctip2 in cortical neurons confers mutually exclusive genetic programs with respect to their targeting [7] , [8] , [24] . Ctip2 dictates a corticofugal fate and is required for the fasciculation and appropriate targeting of these fibres [6] . In contrast, deletion of Satb2 from the neocortex results in the absence of the CC, misrouting of callosal axons towards the internal capsule and an ectopic upregulation of Ctip2 in callosal neurons [7] , [8] . It is interesting to note that although callosal axons fail to cross the midline in Satb2 mutants, not all callosal neurons express Satb2 (ref. 8 ). This suggests that callosal axons may require Satb2 both cell intrinsically and extrinsically. At the same time, some Satb2-positive neurons in deep cortical layers, do not downregulate Ctip2 , and project to the internal capsule [8] . Satb2 was shown to require the transcriptional cofactor Ski in order to repress Ctip2 ; therefore, these Satb2-positive/Ctip2-positive/Ski-negative cells are most likely non-callosal neurons [20] . Data presented here indicate that ectopic upregulation of Ctip2 in callosal neurons is one of the reasons that contribute to the lack of a CC in Satb2 −/− mutants as upon deletion of Ctip2 from the Satb2 −/− cortex, the CC was partially restored. Similar results were also recently reported [7] , [19] . Since the upregulation of Ctip2 in Satb2 −/− mutants is a cell intrinsic effect, the rescue we observed in the Satb2 −/− ; Ctip2 −/− brains is likely to reveal the cell autonomous ability of Satb2 -positive neurons to form the CC [8] . Unc5C and DCC act as receptors for the secreted ligand Netrin1, mediating either a chemorepulsive (Unc5C-DCC together) or a chemoattractive (DCC alone) response [22] , [25] , [26] , [27] . The expression of these two genes is differentially regulated in the neocortex of Satb2 mutants: while Unc5C level is down, DCC is upregulated ( Fig. 9d ). 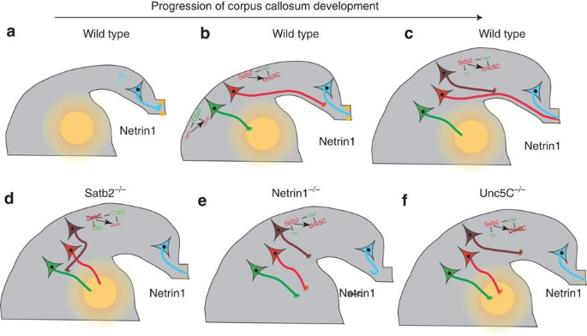Figure 9:Satb2-andCtip2-dependent establishment of cortical connections. (a) During early corticogenesis, cingulate neurons with high DCC expression form the pioneer axons for the CC. These axons respond to midline Netrin1 and are attracted towards the Netrin1 source. (b) Later, when Layer V cells start projecting medially, Satb2 repressesCtip2, thereby promotingUnc5Cexpression. These Unc5C axons are repelled by the Netrin1 source in the internal capsule and thus turn towards the midline. Corticofugally projecting neurons, however, express high Ctip2 and thus repressUnc5C. In addition, the lack of repression ofDCCby Satb2, promotes high DCC levels in these neurons. Thus, these axons are attracted towards the internal capsule (c). Despite expressing high levels of Unc5C and low levels of DCC, upper layer neurons are not dependent on these molecules and instead either follow the deep layer callosal pioneer axons or are dependent on other axon guidance molecules. (d–f) Represent the scenario in theSatb2,Netrin1orUnc5Cmutants, respectively. In each of the mutants, the lack of an Unc5C-Netrin1 interaction causes a misrouting of deep layer callosal axons to subcortical targets. Figure 9: Satb2- and Ctip2 -dependent establishment of cortical connections. ( a ) During early corticogenesis, cingulate neurons with high DCC expression form the pioneer axons for the CC. These axons respond to midline Netrin1 and are attracted towards the Netrin1 source. ( b ) Later, when Layer V cells start projecting medially, Satb2 represses Ctip2 , thereby promoting Unc5C expression. These Unc5C axons are repelled by the Netrin1 source in the internal capsule and thus turn towards the midline. Corticofugally projecting neurons, however, express high Ctip2 and thus repress Unc5C . In addition, the lack of repression of DCC by Satb2, promotes high DCC levels in these neurons. Thus, these axons are attracted towards the internal capsule ( c ). Despite expressing high levels of Unc5C and low levels of DCC, upper layer neurons are not dependent on these molecules and instead either follow the deep layer callosal pioneer axons or are dependent on other axon guidance molecules. ( d – f ) Represent the scenario in the Satb2 , Netrin1 or Unc5C mutants, respectively. In each of the mutants, the lack of an Unc5C-Netrin1 interaction causes a misrouting of deep layer callosal axons to subcortical targets. Full size image We observed that Unc5C expression is regained in Satb2 −/− Ctip2 −/− compound mutants and that Ctip2 acts as a direct transcriptional repressor of Unc5C . Overexpression of Unc5C in Satb2 −/− mutants also leads to a partial restoration of the CC, demonstrating a cell autonomous ability for Unc5C to promote callosal targeting [28] . Srinivasan et al. [19] , independently confirmed this result in a recent publication [7] . This finding at the outset raises the question: If Unc5C is required for CC formation then why are there no obvious defects of the CC observed in Unc5C −/− mutants? Retrograde labelling of subcortically projecting neurons in Unc5C −/− mutants showed that these mutants display an increase in the number of Satb2-positive neurons that project subcortically in these brains ( Fig. 9f ). This indicates that Unc5C is probably required for CC formation only in those neurons that rely on Satb2 cell intrinsically to project callosally. These neurons seem to be early born deep layer neurons but not later born upper layer neurons. Since these axons comprise a smaller population of the CC it is possible that the misrouting of these axons is not easily detected in Unc5C mutants. Unc5C -mediated CC formation is dependent on Unc5C-Netrin1 repulsion. We showed that similar to the Unc5C mutants, Netrin1 mutants had a higher proportion of Satb2-positive cells projecting subcortically compared with wild-type brains. The differences in the proportion of Satb2-positive cells that we observed projecting subcortically in Unc5C −/− when compared with Netrin1 mutants might be due to the different genetic backgrounds of these strains and/or because of the involvement of other Netrin1 receptors such as DCC and Draxin [29] , [30] . It is interesting to note that the Netrin1 mutant is acallosal where as the Unc5C mutant is not. A probable explanation for this could be that although Netrin1 mutants lack a CC, the majority of callosal fibres none the less arrive at the midline but are unable to cross, forming Probst bundles instead [31] . This could be due to the absence of midline Netrin1 expression that otherwise attract DCC expressing cingulate axons, forming the pioneer axons of the CC ( Fig. 9a,e ) [32] . However, in Unc5C mutants, since the midline Netrin1 interaction with DCC-positive cingulate axons is not disrupted, callosal axons cross the midline. Therefore, our data suggest that in Netrin1 mutant and Unc5C −/− -mutant mice, only the callosal fibres that depend on Netrin1–Unc5C interaction, misproject to subcortical targets, whereas neurons that depend on other signalling pathways, continue to project medially towards the midline, where in the Unc5C −/− brains they cross the midline but in the Netrin1 -mutant brains they stall at the midline ( Supplementary Table 1 ). Further, Unc5C- expressing cortical neurons are not repelled by midline Netrin1 probably because at late embryonic stages (E16.5 onwards) the expression level of Netrin1 in the midline is very low as compared with the expression in the basal ganglia [21] , [32] and axons of later born neurons do not require midline Netrin1 to form the CC [32] . In addition, we observed that DCC was upregulated in the absence of Satb2 ( Fig. 9d ). We hypothesized that due to DCC-Netrin1 attraction and the absence of Unc5C-Netrin1-mediated repulsion in Satb2 mutants, callosal fibres that are normally repelled by Netrin1 in the internal capsule are now attracted and hence project subcortically. Interestingly, we found that downregulation of DCC by electroporation of DCC shRNA in Satb2 −/− mice, resulted in a partial rescue of the CC while the DCC mutant displays an acallosal phenotype [22] . This apparent discrepancy could probably again be explained by the fact that although the DCC mutant lacks a CC, cortical axons navigate towards the midline but fail to cross the midline, forming Probst bundles instead [22] . As DCC -positive cingulate axons act as pioneers for the CC, the lack of neocortical callosal midline crossing in DCC knockout animals therefore appears to be due to a secondary defect. In contrast to both the Netrin1 and DCC mutant, in the Satb2 mutant, the acallosal phenotype is not restricted to the absence of callosal midline crossing, but occurs because of the absence of any neocortical axons navigating medially ( Supplementary Table 1 ). Satb2 mutants do not display Probst bundles. All the axons are routed towards the internal capsule and anterior commissure [7] , [8] . Overexpression of Unc5C or downregulation of DCC , in Satb2 −/− brains results in a subset of neurons projecting medially, which can be seen as a clear bundle of axons leaving the electroporated region and approaching the midline. Hence it is not just the midline crossing of these axons that is significant, but more so the choice to project interhemispherically and not in the corticofugal direction. Although we have not been able to detect any neocortical axons forming the CC in our Satb2 mutant, Alcamo et al. [7] reported that their Satb2 mutant has a severely reduced callosum. These few fibres that remain in the Satb2 mutant could be attributed to the presence of DCC -positive cingulate axons that project interhemispherically through the CC that maybe unaffected in the Satb2 mutant ( Fig. 9d ). A simultaneous co-electroporation of Unc5C together with DCC shRNA did not result in a more profound rescue of the CC. Instead, we observed that there was no rescue at all. This is a surprising result indicating that the dosage of Unc5C/DCC in each cell might be critical in deciding the projection fate of cortical projection neurons [33] . Therefore, together, these experiments indicate an important role for Netrin1 , DCC and Unc5C interaction in the trajectory choice made by deep layer cortical axons. We suggest a scenario where the source of Netrin1 in the internal capsule attracts Unc5C-negative/DCC-positive axons while repelling Unc5C-positive/DCC-negative axons. Hence, callosally projecting deep layer neurons require higher levels of Unc5C and lower levels of DCC while on the other hand, low levels of Unc5C and high levels of DCC instruct neurons to project subcortically. It is still not clear how this Netrin1-DCC/Unc5C interaction mechanism functions during the initial steps of axon navigation. We suggest two alternative scenarios. One possibility is that cortical neurons send two axonal branches in two opposite directions, one towards CC and the other towards the internal capsule. The presence of such dual projections in early neocortical development has been reported previously [24] , [34] . Here, Unc5C-positive/DCC-negative neurons would retract the lateral branch after arrival at the Netrin1 source in the internal capsule and stabilize the callosal branch. Unc5C-negative/DCC-positive neurons would retract the callosal branch and stabilize their subcortical branch. A second alternative scenario is that all early cortical neurons send their axons towards the internal capsule, but upon reaching the vicinity of a Netrin1 source, Unc5C-positive/DCC-negative neurons would retract these axons and develop an independent callosal branch. Further studies using live cell imaging would be required to address this issue. Our data strongly indicates that the control of Satb2 and Ctip2 over callosal and corticofugal fate specification is dependent on Unc5C and DCC only with respect to deep layer neurons as none of the rescue experiments performed at E14.5 lead to the formation of a CC. Second, the DiI experiments on Unc5C and Netrin1 mutants predominantly labelled deep layer neurons and thus the differences that we report here are most likely a reflection of the misrouting of deep layer Satb2-positive neurons. Electroporation of Satb2 into the Satb2 −/− brain could as well not rescue the entire acallosal phenotype in these mice, and was effective in rescuing only early born, deep layer, callosal projections. This clearly shows that the potential of each individual Satb2-positive cell to project callosally is highly limited and requires a supportive environment. Hence, it is likely that deep layer neurons act in a cell autonomous manner in deciding between callosal and subcortical fates and that later born Satb2-positive cells are dependent on other mechanisms for correct path finding. Mouse mutants All mouse experiments were carried out in compliance with German law and were approved by the Bezirksregierung Braunschweig and the University of Queensland animal ethics committee. The Satb2-, Ctip2- , Unc5C- and Netrin-1 -mutant mice were generated as described previously [12] , [13] , [35] , [36] . The day of vaginal plug was considered embryonic day (E) 0.5. Wild-type mice used were from a NMRI background. Both male and female embryos were used for the study. Data analysis Data was analysed using Excel or GraphPad Prism. Student’s t -test was used for determining statistical significance. Outgrowth assay Satb2Cre;Rosa flox stop lacZ mice were time-mated (E13 or E17) and pregnant dams were anesthetized with 100 mg kg −1 sodium pentobarbitone, and placed on a heating pad. Embryos were removed and placed in Leibovitz’s L-15 medium (Invitrogen), the brain was removed, and the neocortex dissected. Explants and collagen gels were prepared and cultured exactly as described earlier [32] . Explants displaying poor growth (those below one standard deviation (s.d.) of the mean level of outgrowth for all experiments across all conditions) were eliminated from the experiment. Each explant was stained with TuJ1 IHC as previously described [32] and imaged using a Zeiss upright microscope equipped with an Apotome optical sectioning device. Digital images were analysed using a Matlab (The Mathworks) programme to define a line through the centre of the explant (centre of mass of pixels representing the explant body). The number of pixels representing neurites on either side of this line was then counted (values U and D, respectively). ‘Outgrowth’ was defined as total neurite pixels (U+D) divided by the total number of pixels representing the neurite body [37] , [38] . A total of 46–139 explants per condition were pooled across four experiments and the amount of outgrowth analysed using an unpaired two-tailed Student’s t -test. Data are presented as average values±standard error of the mean (s.e.m.). Tissue processing and IHC Brains were dissected and washed in ice-cold phosphate-buffered saline (PBS) and fixed overnight with 4% paraformaldehyde (wt/vol) followed by treatment with cryo-preservant sucrose and embedding in TissueTek or were processed for vibratome sectioning by embedding in 4% agarose (Applichem). Accordingly, (10 m thick coronal were cut on a cryostat or 80 μm thick on a vibratome. All sections were blocked for 1 h at 24 °C with a solution of 0.1% Triton X-100 (vol/vol) and 2% BSA (wt/vol) in PBS. This was followed by application of the primary antibodies. All antibodies were incubated overnight at 4 °C. Alexa (Molecular Probes) or Dylight (Jackson Immunoresearch) Fluor–tagged secondary antibodies were used at a dilution of 1:500 for 1 h at 24 °C. All sections were mounted in fluorescent mounting medium (DakoCytomation, s3023). The blocking solution used for DiI-labelled sections was 2% BSA in PBS and did not contain any detergent. Primary antibodies used for IHC We used antibodies against GFP (goat, Rockland, 600-202-215, 1:500), Ctip2 (rat, Abcam, ab18465 1:200), DCC (1:100, a kind gift from Dr Helen Cooper), Unc5C (rabbit, self-generated, 1:300), Satb2 (rabbit, self-generated, 1:1,000), L1 (rat, Millipore, MAB5272, 1:150), Calretinin (rabbit, 1:1,000, Swant) and glial fibrillary acidic protein (mouse, 1:500, Sigma). DiI labelling and quantification After fixation in 4% PFA ( Unc5C -mutant brains used for the labelling were fixed for 8 h while the Netrin1 -mutant brains used for the labelling were fixed for more than 3 years), single crystals of 1,1′-dioctadecyl-3,3,3′,3′-tetramethylindocarbocyanine perchlorate (DiI, Molecular probes) were placed with a stainless steel electrode into the cerebral peduncle of the brains. After DiI placement, brains were kept for 2 weeks at 37 °C in PBS with 0.1% sodium azide in the dark. After incubation for the stipulated time, brains were embedded in 4% agarose and sectioned into 80-μm thick sections using a vibratome. Sections were counterstained with Hoechst (Sigma) and mounted in PBS. Alernatively, sections were processed for immunostaining with Satb2. No detergent was used for staining DiI-labelled sections. Images were procured on a Leica SL/SP2 confocal microscope and counting was done manually. Statistics was done using R and Microsoft excel. Graphs were made on GraphPad prism 5. Data are presented as average values±s.d. In Utero electroporation This procedure was carried out as described before [39] . Briefly, pregnant females were anesthetized using Isoflurane inhalation. Temgesic was administered subcutaneously as a painkiller. A 30-mm incision was made into the skin and then the abdominal wall along the midline. Carefully, embryos from either side of the uterine wall were pulled out. Embryos were continuously bathed with a warm solution of 1 × PBS supplemented with penicillin (1,000 units ml −1 )–streptomycin (1,000 μg ml −1 ) to minimize chances of infection. The plasmid solution was injected into one or both lateral ventricles with the help of a picospritzer. Electroporation was carried out by applying six electric pulses of 35 V each, 50 ms duration and 950 ms interval. The animals were allowed to recover and then returned to their cage and kept under observation. At the stage of harvest, the brains were isolated and checked for fluorescence. The brains were then fixed in 4% PFA overnight and embedded in 4% agarose (Applichem) for sectioning using a vibratome. Data are presented as average values±s.e.m. Plasmids The Unc5C, Satb2 , and Ski overexpression plasmids were a kind gift from Dr Frank Polleux, Dr Nenad Sestan and Dr Suzana Atanasoski, respectively. Dr Handjantonakis and Dr Leid kindly provided the CAG-venus-GFP and the pCMV-Ctip2 overexpression plasmid, respectively. The pCAG-Ctip2 overexpression plasmid was cloned by polymerase chain reaction (PCR) from first strand mouse E17.5 cDNA and inserted into the EcoR1-Not1 sites of pCAG. The insert was verified by sequencing. The DCC shRNAs used were purchased from GeneCopoeia. The four different target sequences used were aagccggatgaaggacttt ( DCC shRNA1), agagaccatccaacgtaat ( DCC shRNA2), ttgtcgcctacaatgagtg ( DCC shRNA3), agcagcggtactattccat ( DCC shRNA4). Scrambled shRNA with an unrelated RNA sequence was used. The following primers were used for cloning the Unc5C and DCC RNA probes: Unc5C1 fwd 5′-TCGAATTCGCCGCCACCATGAGGAAAGGTCTGAGGGCGACAG-3′ Unc5C1 rev 5′-AGAGAGTTGAAGGTACCAAATGCTGTGCA-3′ Unc5C2 fwd 5′-TGCACAGCATTTGGTACCTTCAACTCTCT-3′ Unc5C2 rev 5′-TACCCGGGAATACTGTCCTTCTGCTGCCAAGGA-3′ DCC fwd 5′-CCCGATCTTTGGATACATCATGAAG-3′ DCC rev 5′-TCAAAAGGCAGACCCTGTGATGGCGTT-3′. The PCR products were cloned into pGEMT (Promega) and transcribed with T7/Sp6 promoters to generate the RNA probes. In situ hybridization and combined IF-FISH Chromogenic in situ hybridization was performed on overnight fixed tissue samples. Tissues were sectioned with a cryostat at 14–16 μm thickness. Subsequently, the tissue was post-fixed for 15 min in 4% PFA, followed by two PBS washes. The tissue was then treated with Proteinase K for 3 min at room temperature in order to permeabilize the tissue. This step was omitted for the IF-FISH protocol and was instead substituted with a 25-minute incubation in 2 × SSC pH 7.0 (ref. 40 ). Following this, the tissue was either washed in PBS with glycine (to stop the proteinase K reaction) or PBS (IF-FISH). The tissue was then pretreated with the pre-hybridization buffer (50% formamide, 5 × SSC pH 7.0, 2.5 M EDTA, 0.1% Tween-20, 0.15% CHAPS, 0.1 mg ml −1 Heparin, 100 μg ml −1 yeast tRNA, 50 μg ml −1 salmon sperm DNA, 1 × Denhardt’s solution) for 2 h at 65 °C. Following this, the probe was applied and incubated overnight at 65 °C. The following day, the tissue was treated with RNaseA for 30 min at 37 °C, washed with 2 × SSC pH 4.5/50% formamide at 65 °C and then with KTBT (100 mM NaCl, 50 mM Tris–Hcl pH 7.5, 10 mM KCl, 1% Triton X-100). The tissue was then blocked in 20% sheep serum and then incubated overnight with sheep anti-DIG (Roche, 1:1,000) antibody. For the IF-FISH, antibodies against Satb2 and Ctip2 were also included. The following day, the tissue was washed in KTBT and NTMT (50 mM NaCl, 100 mM Tris–HCl pH 9.5, 50 mM MgCl 2, 0.5% Tween-20). The reaction was developed by adding substrate NBT/BCIP (Roche, chromogenic) or Fast Red (Abcam, IF-FISH). Upon reaching the appropriate signal intensity, for the IF-FISH, the sections were washed in PBS and stained with appropriate secondary antibodies. Slice culture and Bead implantation We cut 200–250-μm thick sections of E16.5 Unc5C or EGFP electroporated brains using a vibratome and cultured them on cell culture inserts (1-ct pore size, BD Biosciences) according to the protocol described previously [41] , [42] . The slices were cultured in a medium consisting of complete Hank's Balanced Salt Solution, basal medium Eagle, 20 mM D -glucose, 1 mM L -glutamine, penicillin (100 U ml −1 ), streptomycin (0.1 mg ml −l ), N2 supplement (100 μ, per 12.5 ml) and 10% heat-inactivated horse serum (vol/vol). Agarose beads (Affi-gel Blue gel, Bio-Rad Laboratories) were washed three times with sterile water and four times with PBS. For coating the beads with Netrin1, 20 μl of bead solution was mixed with 10 μl of a Netrin1 solution (250 ng μg −1 R&D Biosciences) and incubated overnight at 4 °C. BSA-coated beads were used as a control for which 20 μl of bead solution was mixed with 20 μl of BSA (1 mg ml −l ). Before placing the beads on the slices, they were washed with PBS and then resuspended in 100 μl. of slice culture medium. Using a mouth pipette, the beads of the desired size were picked and placed over the midline in the region where the CC crosses. The cultured slices were immunostained (see above) after 3 days. Chromatin immunoprecipitation The ChIP IT express kit (Active Motif) was used for performing the ChIP assay, according to the manufacturer’s instructions. Rat monoclonal anti-Ctip2 (Abcam), Satb2 (self-generated) and polyclonal anti-rabbit IgG (Active Motif) antibodies were used. The following primers were used for quantitative real time polymerase chain reaction: Unc5C E1 fwd: 5′-ATCAAGCGCAACTCCCTAAA-3′ Unc5C E1 rev: 5′-CTTGCTCACTTGCTCACTCG-3′ Unc5C E2 fwd: 5′-CCCTTGGAGAAAGTGGAGTG-3′ Unc5C E2 rev: 5′-GTGTACGGGGAAGGGAAAC-3′ DCC MAR1 fwd: 5′-TGCACAGCACCTATGATCTTG-3′ DCC MAR1 rev: 5′ AACAGAGGAGTCAGAGCGAAA-3′ DCC MAR2 fwd: 5′-CGCACACACATTATTCTTTTGG-3′ DCC MAR2 rev: 5′-ACTGCCTGGCTCTGTACTCC-3′. Data are presented as average values±s.d. Luciferase Assay The luciferase assay was done in HEK cells. Unc5C putative Ctip2-binding promoter regions were amplified with the following primers: E1Fw: 5′-TTAAGAATTCTTGCCTTCTTTCCCATCT-3′, E1Rv: 5′-TATTGAGGATCCAGTGCTGGGAGGTGTAGCGC-3′, E2Fw: 5′-TTAAGAATTCTCCTCCTCGGAGGCTC-3′, E2Rv: 5′-TATTGAGGATCCTGAGACGCGCAAACAGCCGA-3′. The fragments were cloned into pC1-TK-luciferase vector (Evrogen). E1 and E2 fragments included −842 to −124 nt and −60 to +65 nt of the Unc5C 5′-flanking promoter region, respectively. Lipofectamine 2000 (Invitrogen) was used for transfecting cells, according to the manufacturer’s instructions. Transfected cells were analysed 24 h after transfection. Luciferase assays were done using the Dual-Luciferase kit (Promega). A mixture of plasmids coding for renilla luciferase (RL) were used (CMV-RL, TK-RL and SV40-RL; 1:2:10 molar proportions, respectively) to account for variable transfection efficiency. Lumat LB96V reader (Berthold Technologies) was used for reading the assays. Results are shown as Renilla-normalized relative luciferase units (RLUs)±s.d. Data shown is at least from three independent experiments. All P -values were ≤0.05. The following primers were used for cloning the DCC MAR1 and MAR2 regions. The PCR products were initially cloned into pGEMT (promega) and sequence verified. Subsequently, the MAR containing inserts were subcloned into pMCS-GL (Thermoscientific). DCC MAR1 fwd 5′-ACTACCTAGTAGAGGCAGCCACAAG-3′ DCC MAR1 rev 5′-AGGTGAAATTTCCACCAATGTGAAT-3′ DCC MAR2 fwd 5′-AAAATGCTACCCATGTTCCAGAAG-3′ DCC MAR2 rev 5′-ACTGCCTGGCTCTGTACTCCAAATT-3′ Fragments cloned into pMCS-GL were transfected along with pCMV-alkaline phosphatase in COS cells using lipofectamine 2000. Forty-eight hours post transfection, cell media was collected and used for assaying using the secrete–Pair Dual Luminescence assay kit (Genecopoeia). Glomax (promega) was used for reading the plates. Values are represented as Ratio of Gaussia luciferase to alkaline phosphatase luminescence ratio±s.d. Values were collected from three independent experiments, with at least three replicates for each experiment. How to cite this article : Srivatsa, S. et al. Unc5C and DCC act downstream of Ctip2 and Satb2 and contribute to corpus callosum formation. Nat. Commun. 5:3708 doi: 10.1038/ncomms4708 (2014).